Chromokinesin Kid and kinetochore kinesin CENP-E differentially support chromosome congression without end-on attachment to microtubules Chromosome congression is the alignment of chromosomes at the spindle equator, and is a prerequisite for faithful chromosome segregation. Recent data suggest that before kinetochores attach to the end of microtubules (end-on attachment), chromosomes can move along microtubules towards the spindle equator through attachment of kinetochores to the lateral surface of microtubules (lateral attachment). Here we address this mechanism, focusing on the contribution of two mitotic motors, Kid and CENP-E. In cells depleted of Hec1, which is essential for end-on attachment, chromosomes show partial and transient congression. This transient congression is further perturbed by co-depletion of Kid, suggesting its role in chromosome congression. In comparison, CENP-E suppresses chromosome congression, probably by tethering kinetochores to short, unstable microtubules, and works in congression only when microtubules are stabilized. Our results may reflect the differential contributions of Kid and CENP-E in chromosome congression in physiological conditions where stabilized microtubules are becoming increased. In the classic ‘search and capture’ model of chromosome attachment to microtubules during mitosis, chromosome congression occurs as a result of the establishment of bi-orientation [1] , which is the end-on attachment of sister kinetochores to microtubules from opposite spindle poles. However, recent data suggest that chromosome congression can occur in the absence of bi-orientation, and bi-orientation is established at the spindle equator while lateral attachment is converted to end-on attachment [2] , [3] . Congression of laterally attached chromosomes is thought to be achieved by transport along spindle microtubules by CENP-E [2] , [4] , a microtubule plus-end-directed motor of the kinesin-7 family localizing to kinetochores [5] , and polar ejection forces (PEFs) [6] exerted mainly by Kid [7] , [8] , [9] , a chromokinesin of the kinesin-10 family localizing to chromosomes. The relative contribution of these two mechanisms is not clear. A role for CENP-E in chromosome congression was initially reported as a means to facilitate congression of mono-oriented chromosomes, which have formed end-on attachment with only one of the sister kinetochores, along pre-existing kinetochore fibres (microtubule bundles that extend from kinetochores to spindle poles) [4] . It was later found that such anti-poleward chromosome motion could occur even in the absence of kinetochore fibres [2] . The contribution of chromokinesins to chromosome congression was reported for a Kid homologue in Xenopus laevis , using in vitro -assembled spindles [7] , [10] . In contrast, only a minor defect was seen when Kid was depleted in mammalian cells [8] , [9] , [11] , [12] . Here we demonstrate that the role of Kid in chromosome congression becomes apparent when the formation of end-on attachment is suppressed. Surprisingly, CENP-E, in contrast, inhibits chromosome congression in the same situation, and it contributes to the process when microtubules are stabilized. We propose a model in which Kid and CENP-E cooperatively contribute to chromosome congression in physiological conditions, depending on the stability of spindle microtubules. Kid plays a role in chromosome congression We tested the role of Kid and CENP-E in HeLa cells expressing EGFP–CENP-A by observing chromosome alignment when these motors were depleted ( Fig. 1a ). As reported previously, Kid depletion in mammalian cells did not show apparent alignment defects [8] , [9] , [11] , [12] , whereas misaligned chromosomes attaching to the spindle poles were observed in CENP-E-depleted cells [13] , [14] , [15] ( Fig. 1b,c ; Supplementary Fig. 1 ). When both motors were depleted simultaneously, we found more chromosomes failed to align ( Fig. 1b,c ). In addition, when the time spent in each phase of mitosis was quantified, by live cell imaging, prometaphase was longer in Kid-depleted cells compared with control cells ( Fig. 1d,e ), consistent with previous reports [3] , [9] . We also confirmed that CENP-E-depleted cells, with or without Kid depletion, arrested in mitosis [14] , [16] ( Fig. 1d ). These data suggest that Kid plays a role in chromosome congression, which becomes apparent when CENP-E is co-depleted. 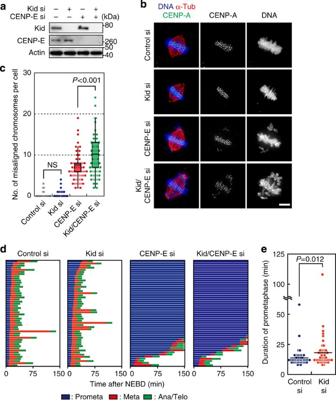Figure 1: Contribution of Kid to chromosome alignment. (a) Depletion of Kid and CENP-E by RNAi. The protein levels were analysed by western blotting with antibodies as indicated. (b) Chromosome alignment in cells depleted of Kid and/or CENP-E. Mitotic HeLa cells expressing EGFP–CENP-A treated with the indicated siRNAs were fixed and stained with anti-GFP (green) and anti-α-tubulin (red). DNA was stained with 4,6-diamidino-2-phenylindole (blue). Scale bar, 5 μm. (c) Number of misaligned chromosomes in Kid- and/or CENP-E-depleted cells. The numbers of misaligned chromosomes per cell are displayed as box and dot plots. The data represent 100 cells for each category. In box plots, the bottom and top of the box show the lower and upper quartile values, respectively. The median is indicated with a bar in the box, and the whiskers denote the range within 1.5 × size of the box.Pvalue was obtained using a Mann–WhitneyU-test. NS, not statistically significant. (d) Duration of mitosis in Kid- and/or CENP-E-depleted cells. HeLa cells expressing EGFP–α-tubulin, EGFP–CENP-A and H2B–mCherry treated with the indicated siRNAs were observed after release from the thymidine block. Duration of prometaphase (prometa: from nuclear envelope breakdown (NEBD) to chromosome alignment; blue), metaphase (meta: from chromosome alignment to anaphase onset; red) or anaphase/telophase (ana/telo: from anaphase onset to chromosome decondensation; green) was indicated. The data represent 50 cells for each category. (e) Duration of prometaphase in Kid-depleted cells. The results indare displayed as dot plots. The median is indicated with a bar.Pvalue was obtained using the Mann–WhitneyU-test. Figure 1: Contribution of Kid to chromosome alignment. ( a ) Depletion of Kid and CENP-E by RNAi. The protein levels were analysed by western blotting with antibodies as indicated. ( b ) Chromosome alignment in cells depleted of Kid and/or CENP-E. Mitotic HeLa cells expressing EGFP–CENP-A treated with the indicated siRNAs were fixed and stained with anti-GFP (green) and anti-α-tubulin (red). DNA was stained with 4,6-diamidino-2-phenylindole (blue). Scale bar, 5 μm. ( c ) Number of misaligned chromosomes in Kid- and/or CENP-E-depleted cells. The numbers of misaligned chromosomes per cell are displayed as box and dot plots. The data represent 100 cells for each category. In box plots, the bottom and top of the box show the lower and upper quartile values, respectively. The median is indicated with a bar in the box, and the whiskers denote the range within 1.5 × size of the box. P value was obtained using a Mann–Whitney U -test. NS, not statistically significant. ( d ) Duration of mitosis in Kid- and/or CENP-E-depleted cells. HeLa cells expressing EGFP–α-tubulin, EGFP–CENP-A and H2B–mCherry treated with the indicated siRNAs were observed after release from the thymidine block. Duration of prometaphase (prometa: from nuclear envelope breakdown (NEBD) to chromosome alignment; blue), metaphase (meta: from chromosome alignment to anaphase onset; red) or anaphase/telophase (ana/telo: from anaphase onset to chromosome decondensation; green) was indicated. The data represent 50 cells for each category. ( e ) Duration of prometaphase in Kid-depleted cells. The results in d are displayed as dot plots. The median is indicated with a bar. P value was obtained using the Mann–Whitney U -test. Full size image Partial chromosome congression in Hec1-depleted cells To investigate the mechanisms of chromosome congression before end-on attachment is formed, we observed cells depleted of Hec1, a component of the Ndc80 complex required for end-on attachment [17] ( Fig. 2b ). We used HeLa cells expressing EGFP–α-tubulin, EGFP–CENP-A and H2B–mCherry to visualize microtubules, kinetochores and chromosomes, respectively, for live cell imaging. Control cells showed clear chromosome congression that resulted in the compaction of the chromosomes on the metaphase plate ( Fig. 2b , 35 min; Supplementary Movie 1 ). Hec1 depletion was assessed by the reduction of its expression to below a detectable level by western blotting (WB) ( Fig. 2a ), and premature anaphase onset due to abrogation of the spindle assembly checkpoint [18] ( Supplementary Fig. 2a ). In spite of the defect in end-on attachment, most chromosomes showed frequent back-and-forth motions parallel to the spindle axis ( Supplementary Movie 2 ), suggesting a connection to spindle microtubules at their lateral surface, as previously reported [2] , [3] . We confirmed that most of the kinetochores in Hec1-depleted cells were laterally attached to microtubules by immunofluorescence (IF) staining ( Supplementary Fig. 2b ). Chromosomes did not properly align on the spindle equator in Hec1-depleted cells, and were eventually distributed randomly around the spindle poles ( Fig. 2b , 35 min; Supplementary Movie 2 ). However, we noticed that, shortly after nuclear envelope breakdown, chromosomes showed a clear tendency to move towards the spindle equator ( Fig. 2b ). Lack of chromosome pulling/pushing forces by end-on-attached microtubules to bi-oriented kinetochores [19] , which keeps chromosomes around the spindle equator, may explain the inefficiency of this partial and transient congression. It may also be explained by the reduction of microtubule density in the middle of the spindle, due to lack of microtubule stabilization by end-on attachment. Next, we observed the contributions of Kid and CENP-E to this partial congression. WB analysis showed that these motor proteins were efficiently depleted ( Fig. 2a ). When we depleted Kid in addition to Hec1, the chromosome movement towards the spindle equator was less clear, and chromosomes were distributed more diffusely along the spindle ( Fig. 2b ; Supplementary Movie 3 ), suggesting that Kid is involved in this partial congression. In contrast, when CENP-E was depleted together with Hec1, chromosomes gathered more tightly around the spindle equator ( Fig. 2b ; Supplementary Movie 4 ). When Hec1, Kid and CENP-E were all depleted together, the congression was impaired, as in Hec1, Kid co-depleted cells ( Fig. 2b ; Supplementary Movie 5 ). These results imply that Kid promotes the partial and transient congression in Hec1-depleted cells, whereas CENP-E suppresses it. 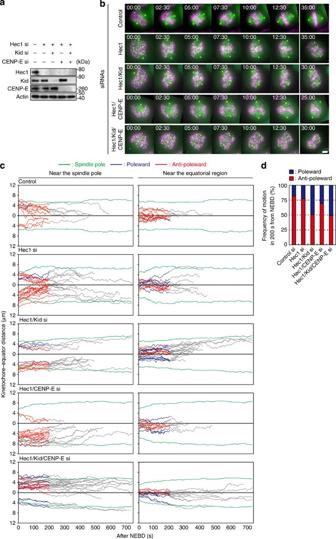Figure 2: Partial and transient chromosome congression in Hec1-depleted cells. (a) Depletion of Hec1, Kid and CENP-E by RNAi. The protein levels were analysed by western blotting with antibodies as indicated. (b) Live imaging of cells depleted of Kid and/or CENP-E together with Hec1. HeLa cells expressing EGFP–α-tubulin, EGFP–CENP-A and H2B–mCherry were treated with the indicated siRNAs and imaged at 5-s intervals, starting from NEBD. Time (min:s) is indicated in the upper left in each panel. Asterisks mark the positions of spindle poles. See alsoSupplementary Movies 1,2,3,4,5. Scale bar, 5 μm. (c) Trajectories of kinetochore motion in prometaphase cells. A minimum of 29 EGFP–CENP-A dots in cells shown inbwere tracked for a maximum of 740 s after NEBD. The distance between spindle poles and the spindle equator is shown as green lines. For clarity, kinetochores are categorized as being closer to either spindle poles or the spindle equator at NEBD, and shown separately. The distance between kinetochores and the spindle equator is shown, classified as either poleward (blue lines) or anti-poleward motion (red lines), according to the net direction of kinetochore motion during the first 200 s. Trajectories of all the kinetochores after 200 s are shown by grey lines. (d) Frequencies of poleward and anti-poleward motions. The percentages of poleward (blue) and anti-poleward motions (red) of kinetochores in cells shown incandSupplementary Fig. 3a(11 cells in total for each condition) are shown. Figure 2: Partial and transient chromosome congression in Hec1-depleted cells. ( a ) Depletion of Hec1, Kid and CENP-E by RNAi. The protein levels were analysed by western blotting with antibodies as indicated. ( b ) Live imaging of cells depleted of Kid and/or CENP-E together with Hec1. HeLa cells expressing EGFP–α-tubulin, EGFP–CENP-A and H2B–mCherry were treated with the indicated siRNAs and imaged at 5-s intervals, starting from NEBD. Time (min:s) is indicated in the upper left in each panel. Asterisks mark the positions of spindle poles. See also Supplementary Movies 1 , 2 , 3 , 4 , 5 . Scale bar, 5 μm. ( c ) Trajectories of kinetochore motion in prometaphase cells. A minimum of 29 EGFP–CENP-A dots in cells shown in b were tracked for a maximum of 740 s after NEBD. The distance between spindle poles and the spindle equator is shown as green lines. For clarity, kinetochores are categorized as being closer to either spindle poles or the spindle equator at NEBD, and shown separately. The distance between kinetochores and the spindle equator is shown, classified as either poleward (blue lines) or anti-poleward motion (red lines), according to the net direction of kinetochore motion during the first 200 s. Trajectories of all the kinetochores after 200 s are shown by grey lines. ( d ) Frequencies of poleward and anti-poleward motions. The percentages of poleward (blue) and anti-poleward motions (red) of kinetochores in cells shown in c and Supplementary Fig. 3a (11 cells in total for each condition) are shown. Full size image To see the effect of Kid or CENP-E depletion on this partial congression in more detail, we tracked individual kinetochores observed by live cell imaging. Trajectories of kinetochores in Hec1-depleted cells showed that the majority of the kinetochores initially moved towards the spindle equator in a similar manner to that of control cells ( Fig. 2c ; Supplementary Fig. 3a ). However, a fraction of kinetochores either did not reach, or left, the spindle equator, resulting in inefficient congression. In Hec1, Kid co-depleted cells, kinetochore motion towards the spindle equator was not apparent and most of the kinetochores neither reached nor stayed around the spindle equator ( Fig. 2c ; Supplementary Fig. 3a ). Cells depleted of Kid alone showed kinetochore motion towards the spindle equator ( Supplementary Fig. 3b ). In Hec1, CENP-E co-depleted cells, many kinetochores reached and stayed close to the spindle equator ( Fig. 2c ; Supplementary Fig. 3a ). Kinetochores in Hec1, Kid, CENP-E co-depleted cells behaved similarly to Hec1, Kid co-depleted cells ( Fig. 2c ; Supplementary Fig. 3a ). Next we assessed the net direction of kinetochore motion along the spindle axis during the first 200 s after nuclear envelope breakdown. As shown in Fig. 2d , anti-poleward motion predominated in Hec1-depleted cells, as in control cells. The frequency of anti-poleward motion was reduced in Kid, Hec1 co-depleted cells, indicating a role for Kid in this partial congression. Hec1, CENP-E co-depleted cells showed a frequency of anti-poleward motion similar to that in Hec1-depleted cells ( Fig. 2d ). In Hec1, Kid, CENP-E co-depleted cells, anti-poleward motion decreased as in Hec1, Kid co-depleted cells ( Fig. 2d ). These analyses strengthen our idea that Kid plays a major role in the partial and transient congression in Hec1-depleted cells while CENP-E plays an inhibitory role. Roles of Kid and CENP-E in kinetochore distribution In live cell imaging, the number of kinetochores that can be followed was limited due to poor resolution of images as a result of off-axis illumination. Therefore, we used fixed samples to allow us to observe the distribution of all the kinetochores on the spindle in Hec1-depleted cells. Cells were released from thymidine treatment and fixed at a time when early mitotic cells were enriched ( Fig. 3a ). We then measured the distance between kinetochores and the spindle equator, and plotted the relative distance along the half spindle ( Fig. 3b ; distance between the spindle equator and a spindle pole was adjusted to 10). This value was 3.07±2.57 (mean±s.d., n =1,078) in Hec1-depleted cells, which was larger than that in control metaphase cells (1.33±0.98 ( n =952); Fig. 3b ). The relative kinetochore to spindle equator distance was even greater in Hec1, Kid co-depleted cells (3.65±2.41 ( n =1,067); Fig. 3b ). In comparison, the value was smaller in Hec1, CENP-E co-depleted cells (2.33±1.98 ( n =1,072); Fig. 3b ). When Hec1, Kid and CENP-E were all depleted together, the value was similar to that in Hec1, Kid co-depleted cells (3.86±2.50 ( n =1,080); Fig. 3b ). We confirmed that the difference in the relative kinetochore distribution in the spindle was not due to a change in the spindle length. Although Hec1 depletion caused spindle elongation, additional Kid and/or CENP-E depletion did not change the spindle length further ( Supplementary Fig. 4a ). These findings correlate well with the live cell imaging results, and show that kinetochore distribution examined in fixed samples can be a useful index to judge the efficiency of chromosome congression. To see whether these findings are applicable to other cell lines, we observed kinetochore distribution in RPE-1 cells (non-transformed cells) and HCT116 cells (near-diploid cancer cells) in the same conditions as for the, highly aneuploid, HeLa cells. As shown in Supplementary Fig. 4b–d , both cells showed similar results to HeLa cells; Kid depletion increased, and CENP-E depletion reduced the relative kinetochore to spindle equator distance in Hec1-depleted cells. These results confirmed the idea that Kid and CENP-E play antagonistic roles in the partial chromosome congression seen in Hec1-depleted cells. 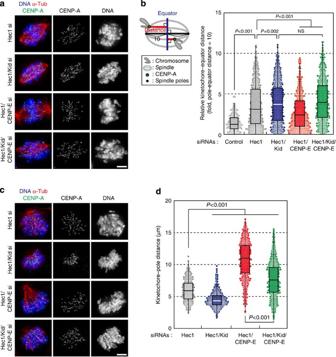Figure 3: Kinetochore distribution in cells depleted of Kid and/or CENP-E together with Hec1. (a) Chromosome distribution in cells depleted of Kid and/or CENP-E together with Hec1. Mitotic HeLa cells expressing EGFP–CENP-A treated with the indicated siRNAs were fixed 10 h after release from the thymidine block, and stained with anti-GFP (green) and anti-α-tubulin (red). DNA was stained with 4,6-diamidino-2-phenylindole (DAPI) (blue). Scale bar, 5 μm. (b) Relative distance between kinetochores and the spindle equator. The relative kinetochore to spindle equator distance was measured as shown in the left cartoon and displayed as inFig. 1c. The data represent a minimum of 952 EGFP–CENP-A dots from 10 cells for each category.Pvalues were obtained using the Mann–WhitneyU-test. NS, not statistically significant. (c) Chromosome distribution in cells with monopolar spindles depleted of Kid and/or CENP-E together with Hec1. Mitotic HeLa cells expressing EGFP–CENP-A treated with indicated siRNAs were treated with 1 μM Eg5 inhibitor lll for 2 h, 9 h after release from the thymidine block. Cells were fixed and stained with anti-GFP (green) and anti-α-tubulin (red). DNA was stained with DAPI (blue). Scale bar, 5 μm. (d) Kinetochore–spindle pole distance. The graph shows the distance between kinetochores to the mid-point between spindle poles incand is displayed as inFig. 1c. The data represent a minimum of 481 EGFP–CENP-A dots from five cells for each category.Pvalue was obtained by the Mann–WhitneyU-test. Figure 3: Kinetochore distribution in cells depleted of Kid and/or CENP-E together with Hec1. ( a ) Chromosome distribution in cells depleted of Kid and/or CENP-E together with Hec1. Mitotic HeLa cells expressing EGFP–CENP-A treated with the indicated siRNAs were fixed 10 h after release from the thymidine block, and stained with anti-GFP (green) and anti-α-tubulin (red). DNA was stained with 4,6-diamidino-2-phenylindole (DAPI) (blue). Scale bar, 5 μm. ( b ) Relative distance between kinetochores and the spindle equator. The relative kinetochore to spindle equator distance was measured as shown in the left cartoon and displayed as in Fig. 1c . The data represent a minimum of 952 EGFP–CENP-A dots from 10 cells for each category. P values were obtained using the Mann–Whitney U -test. NS, not statistically significant. ( c ) Chromosome distribution in cells with monopolar spindles depleted of Kid and/or CENP-E together with Hec1. Mitotic HeLa cells expressing EGFP–CENP-A treated with indicated siRNAs were treated with 1 μM Eg5 inhibitor lll for 2 h, 9 h after release from the thymidine block. Cells were fixed and stained with anti-GFP (green) and anti-α-tubulin (red). DNA was stained with DAPI (blue). Scale bar, 5 μm. ( d ) Kinetochore–spindle pole distance. The graph shows the distance between kinetochores to the mid-point between spindle poles in c and is displayed as in Fig. 1c . The data represent a minimum of 481 EGFP–CENP-A dots from five cells for each category. P value was obtained by the Mann–Whitney U -test. Full size image To further validate these results, and to exclude the effects of the presence of anti-parallel microtubules, we observed kinetochore distribution in a monopolar spindle ( Fig. 3c ). Cells were treated with an inhibitor of the kinesin-5 motor, Eg5 (ref. 20 ), which is required for bipolarity of the spindle, and the distance between kinetochores and the mid-point of clustered spindle poles was measured ( Fig. 3d ). Compared with Hec1-depleted cells (5.94±1.66 μm ( n =481)), kinetochores were closer to spindle poles in Hec1, Kid co-depleted cells (4.56±1.22 μm ( n =554)). In Hec1, CENP-E co-depleted cells, the kinetochore to spindle pole distance was longer (10.78±2.88 μm ( n =737); Fig. 3d ), and kinetochores localized close to the microtubule plus ends in monopolar spindles. The distance was shortened when Kid was depleted together with Hec1 and CENP-E (7.68±2.71 μm ( n =792); Fig. 3d ). These results are consistent with the results in bipolar spindles, and strongly support the idea that Kid is involved in the chromosome congression in Hec1-depleted cells, while CENP-E suppresses it. Roles of motor activities in kinetochore distribution Next we assessed whether the motor activities are required for the role of Kid and CENP-E in the kinetochore distribution seen in Hec1-depeleted cells. First, either RNA interference (RNAi)-resistant wild type, or a rigor mutant of Kid, each tagged with a myc-epitope, was expressed in cells depleted of Kid and Hec1 ( Supplementary Fig. 5a ). Expression of myc–Kid varied considerably between cells, and we selected cells expressing exogenous Kid at similar levels to that of the endogenous protein ( Fig. 4a ; Supplementary Fig. 5b ); excessive expression caused severe defects in spindle organization ( Supplementary Fig. 5c ). Wild-type Kid restored the relative kinetochore to spindle equator distance (from 4.36±2.80 ( n =380) to 3.29±2.52 ( n =271); Fig. 4b ) to that comparable to Hec1-depleted cells (3.15±2.13 ( n =366)), confirming the specificity of the phenotype, but a Kid rigor mutant could not rescue the increased distance in Kid-depleted cells (5.21±3.63 ( n =361); Fig. 4b ), suggesting that motor activity is required for the role of Kid to locate kinetochores close to the spindle equator in Hec1-depleted cells. Next, either wild-type or a rigor mutant of CENP-E, tagged with a mycGFP-epitope, was expressed in cells depleted of CENP-E, by short interfering RNA (siRNA) targeting the 3′ untranslated region (UTR), together with Hec1 ( Supplementary Fig. 5a ). As for Kid, above, we selected cells expressing exogenous CENP-E at similar levels to the endogenous protein ( Fig. 4a ; Supplementary Fig. 5d ); again, excessive expression caused severe defects in spindle organization ( Supplementary Fig. 5e ). Wild-type CENP-E reverted the reduction in the relative kinetochore to spindle equator distance (from 2.77±2.15 ( n =406) to 4.21±2.72 ( n =430); Fig. 4b ), as expected. Intriguingly, a CENP-E rigor mutant further increased the distance (5.66±3.68 ( n =397); Fig. 4b ). As the CENP-E rigor mutant is assumed to be immobilized on microtubules [21] , this result suggests that the mutant keeps kinetochores away from the spindle equator by tethering kinetochores to microtubules. We also checked the result using a CENP-E inhibitor, GSK923295 (ref. 22 ), which locks CENP-E in a rigor, microtubule-bound state. We confirmed the efficacy of the inhibitor by observing the appearance of misaligned chromosomes around spindle poles, and found that, in the presence of the inhibitor, CENP-E localized to kinetochores in Hec1-depleted cells ( Fig. 4c ). As shown in Fig. 4d , CENP-E inhibition increased the kinetochore to spindle equator distance similarly to the expression of the rigor mutant, confirming that CENP-E tightly bound to microtubules locates kinetochores away from the spindle equator. 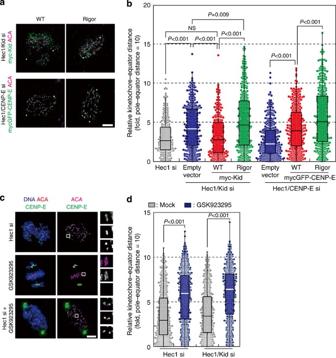Figure 4: Roles of Kid and CENP-E motor activities for the kinetochore distribution in Hec1-depleted cells. (a) Cells expressing Kid or CENP-E constructs. Hec1, Kid co-depleted cells expressing myc–Kid constructs, and CENP-E, Hec1 co-depleted cells expressing mycGFP–CENP-E constructs were fixed 10 h after release from the thymidine block, and stained with anti-myc or anti-GFP (green), and anti-centromeric antigen (ACA; magenta). Asterisks indicate the positions of spindle poles. Scale bar, 5 μm. (b) Relative distance between kinetochores and the spindle equator. The relative kinetochore to spindle equator distance was measured and displayed as inFig. 3b. The data represent a minimum of 271 ACA dots from five cells expressing the rescue constructs.Pvalue was obtained using the Mann–WhitneyU-test. NS, not statistically significant. (c) Localization of CENP-E in the presence of GSK923295. HeLa cells with or without Hec1 depletion were treated with 200 nM CENP-E inhibitor (GSK923295) for 2 h, 9 h after release from the thymidine block. Cells were fixed and stained with anti-CENP-E (green) and ACA (magenta). DNA was stained with DAPI (blue). Note that CENP-E decreases on aligned kinetochores (middle panels). Scale bar, 5 μm. (d) Relative distance between kinetochores and the spindle equator. The relative kinetochore to spindle equator distance in cells treated with indicated siRNAs in the presence or absence of GSK923295 was measured and displayed as inFig. 3b. The data represent a minimum of 951 ACA dots from 10 cells for each category.Pvalues were obtained using the Mann–WhitneyU-test. Figure 4: Roles of Kid and CENP-E motor activities for the kinetochore distribution in Hec1-depleted cells. ( a ) Cells expressing Kid or CENP-E constructs. Hec1, Kid co-depleted cells expressing myc–Kid constructs, and CENP-E, Hec1 co-depleted cells expressing mycGFP–CENP-E constructs were fixed 10 h after release from the thymidine block, and stained with anti-myc or anti-GFP (green), and anti-centromeric antigen (ACA; magenta). Asterisks indicate the positions of spindle poles. Scale bar, 5 μm. ( b ) Relative distance between kinetochores and the spindle equator. The relative kinetochore to spindle equator distance was measured and displayed as in Fig. 3b . The data represent a minimum of 271 ACA dots from five cells expressing the rescue constructs. P value was obtained using the Mann–Whitney U -test. NS, not statistically significant. ( c ) Localization of CENP-E in the presence of GSK923295. HeLa cells with or without Hec1 depletion were treated with 200 nM CENP-E inhibitor (GSK923295) for 2 h, 9 h after release from the thymidine block. Cells were fixed and stained with anti-CENP-E (green) and ACA (magenta). DNA was stained with DAPI (blue). Note that CENP-E decreases on aligned kinetochores (middle panels). Scale bar, 5 μm. ( d ) Relative distance between kinetochores and the spindle equator. The relative kinetochore to spindle equator distance in cells treated with indicated siRNAs in the presence or absence of GSK923295 was measured and displayed as in Fig. 3b . The data represent a minimum of 951 ACA dots from 10 cells for each category. P values were obtained using the Mann–Whitney U -test. Full size image CENP-E works for congression on stabilized microtubules Why does CENP-E suppress chromosome congression in Hec1-depleted cells when it is known to function in chromosome congression along kinetochore fibres [4] ? In Hec1-depleted cells, spindle microtubules are unstable due to lack of kinetochore fibres, which may explain the different contributions of CENP-E to chromosome congression. To test this, we examined kinetochore distribution when microtubules were stabilized by depletion of MCAK [23] , a microtubule depolymerizing kinesin of the kinesin-13 family ( Fig. 5a ; Supplementary Fig. 6a ). Microtubule stabilization by MCAK depletion resulted in a remaining tubulin intensity in the middle of the spindle after cold treatment ( Fig. 5c,d ). The relative kinetochore to spindle equator distance was decreased by MCAK depletion in Hec1-depleted cells (from 3.09±2.56 ( n =1,107) to 2.24±2.10 ( n =968)), suggesting that microtubule stabilization promotes chromosome congression in Hec1-depleted cells ( Fig. 5a,b ). The distance in Hec1, Kid co-depleted cells was also reduced by MCAK depletion (from 3.56±2.37 ( n =1,019) to 2.68±2.26 ( n =1,048); Fig. 5a,b ). However, MCAK depletion did not change the distance in Hec1, CENP-E co-depleted cells (from 2.40±2.29 ( n =1,040) to 2.32±2.17 ( n =1,069); Fig. 5a,b ). These data can best be explained by a model, in which CENP-E contributes to chromosome congression in Hec1-depleted cells in the presence of stabilized microtubules and, in its absence, Kid compensates for the function of CENP-E. CENP-E is a slow, processive motor [21] that has a reduced affinity for microtubules after phosphorylation by Aurora kinases [24] , which makes the motor work more efficiently on bundled microtubules, for example, kinetochore fibres, which allow a rapid rebinding of the motor to adjacent microtubules. It is plausible that MCAK depletion increases the microtubule density as well as the population of long microtubules, allowing efficient walking of CENP-E along microtubules towards the spindle equator. Alternatively, CENP-E is also known to work as a microtubule tip-tracker, using both its motor and tail domains [25] . Therefore, CENP-E at the tips of short, unstable microtubules in Hec1-depleted cells may suppress chromosome motion towards the spindle equator by tethering kinetochores to these microtubule tips. In addition, chromosomes close to the spindle equator may be pulled back to the spindle poles by CENP-E at the tips of shrinking microtubules. Compared with CENP-E, Kid is a fast, but low processive motor [26] , which is probably why it works irrespective of microtubule stability. In a previous study, it was reported that chromosome alignment in cells depleted of Nuf2, a component of the Ndc80 complex, was significantly restored by co-depletion of HSET [2] , a minus-end-directed motor belonging to the kinesin-14 family [27] , [28] . We confirmed that the kinetochore to spindle equator distance was decreased by co-depletion of HSET in Hec1-depleted cells ( Fig. 5a,b ; Supplementary Fig. 6a ). Also, HSET depletion increased the microtubule stability around the spindle equator in Hec1-depleted cells, as determined by the sensitivity of microtubules to cold treatment ( Fig. 5c,d ). The microtubule stabilization by HSET depletion may explain the improvement of chromosome congression in Hec1-depleted cells by promoting the function of CENP-E. In agreement with this idea, the kinetochore to spindle equator distance was also decreased by HSET depletion in Kid, Hec1 co-depleted cells ( Fig. 5b ). This is consistent with a previous report that CENP-E is responsible for chromosome congression in Nuf2, HSET co-depleted cells [2] . In contrast, HSET depletion increased the distance in CENP-E, Hec1 co-depleted cells ( Fig. 5b ), suggesting that Kid negatively affected the chromosome congression in Hec1-depleted cells in this situation. HSET is known to crosslink, and slide between, parallel microtubules in mitosis [28] . HSET depletion may cause the increase in microtubule density around the spindle equator due to the defect in microtubule sliding towards spindle poles, as suggested previously [2] . We verified the differences in the microtubule environment caused by MCAK and HSET depletion in Hec1-depleted cells. We quantified α-tubulin intensity to evaluate microtubule mass, and number and intensity of EB1 (a plus-end tracking protein) dots to assess microtubule number and degree of microtubule bundling, respectively ( Fig. 5e–i ). The number of EB1 dots increased by both MCAK and HSET depletion, while α-tubulin intensity increased only after MCAK depletion ( Fig. 5f,g ). Accordingly, HSET depletion caused an increase in the number, but a decrease in the intensity, of EB1 dots relative to the α-tubulin intensity ( Fig. 5h,i ). These results are consistent with the idea that longer microtubules were increased by MCAK depletion, whereas less-bundled overlapping microtubules increased after HSET depletion ( Supplementary Fig. 6b ). Such a difference may distinctively affect the function of Kid, while the increase in microtubule density in the equatorial region improved the function of CENP-E in both cases. As a premise for the discussion above, we excluded the possibility that the difference in the relative kinetochore distribution was due to a change in the spindle length after depletion of MCAK or HSET, by comparing the spindle length in the different conditions ( Supplementary Fig. 6c ). In our measurements, spindle length was comparable between Hec1-depleted cells and Hec1, HSET co-depleted cells ( Supplementary Fig. 6c ), which is in contrast with the previous report that spindle elongation in Nuf2-depleted cells was partially rescued by HSET depletion [28] . This discrepancy can be explained by the timing of observation in mitosis, because we also found the reduction in the spindle length in Hec1, HSET co-depleted cells at a later time point after release from a thymidine block ( Supplementary Fig. 7 ). Overall, these results support the idea that CENP-E contributes to chromosome congression when microtubules are stabilized. 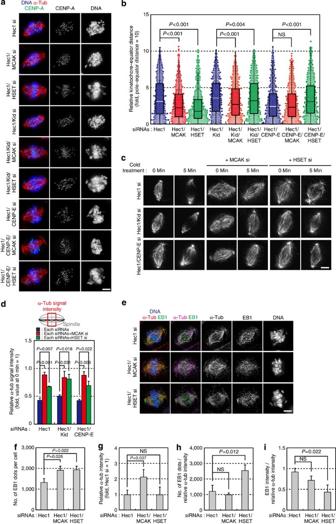Figure 5: Microtubule stabilization promotes the role of CENP-E in chromosome congression in Hec1-depleted cells. (a) Chromosome distribution in cells depleted of Kid, CENP-E, MCAK or HSET together with Hec1. Mitotic HeLa cells expressing EGFP–CENP-A treated with the indicated siRNAs were fixed 10 h after release from the thymidine block, and stained with anti-GFP (green) and anti-α-tubulin (red). DNA was stained with 4,6-diamidino-2-phenylindole (DAPI) (blue). Scale bar, 5 μm. (b) Relative distance between kinetochores and the spindle equator. The relative kinetochore to spindle equator distance was measured and displayed as inFig. 3b. The data represent a minimum of 1019 EGFP–CENP-A dots from 10 cells for each category.Pvalues were obtained using the Mann–WhitneyU-test. NS, not statistically significant. (c) Spindle appearance of cells depleted of Kid, CENP-E, MCAK or HSET together with Hec1 after cold treatment. Mitotic HeLa cells treated with the indicated siRNAs were incubated on ice for 0 or 5 min before fixation and staining with anti-α-tubulin. Scale bar, 5 μm. (d) Quantification of microtubule signals in the middle of the spindle. The α-tubulin signal intensities in the middle region of a three-way split spindle as schematized were measured and the relative values at 5 min on ice are indicated in a bar graph. (e) Distribution of EB1 in cells depleted of MCAK or HSET together with Hec1. Mitotic HeLa cells were stained with anti-EB1 (green) and anti-α-tubulin (magenta). DNA was stained with DAPI (blue). All panels represent a single Z-section. Scale bar, 5 μm. (f) Number of EB1 dots per cell. The graph shows average number of EB1 dots in each cell. (g) Quantification of the microtubule signal per cell. The graph shows relative intensity of α-tubulin signal in each cell. (h,i) The number of EB1 dots (h) and the intensity of EB1 signals (i) were compared after adjustment by relative microtubule signal intensity ing. For the graphs indandf–i, error bars represent the s.d. of three independent experiments measuring 10 cells each.Pvalues were obtained by Student’st-test. NS, not statistically significant. Figure 5: Microtubule stabilization promotes the role of CENP-E in chromosome congression in Hec1-depleted cells. ( a ) Chromosome distribution in cells depleted of Kid, CENP-E, MCAK or HSET together with Hec1. Mitotic HeLa cells expressing EGFP–CENP-A treated with the indicated siRNAs were fixed 10 h after release from the thymidine block, and stained with anti-GFP (green) and anti-α-tubulin (red). DNA was stained with 4,6-diamidino-2-phenylindole (DAPI) (blue). Scale bar, 5 μm. ( b ) Relative distance between kinetochores and the spindle equator. The relative kinetochore to spindle equator distance was measured and displayed as in Fig. 3b . The data represent a minimum of 1019 EGFP–CENP-A dots from 10 cells for each category. P values were obtained using the Mann–Whitney U -test. NS, not statistically significant. ( c ) Spindle appearance of cells depleted of Kid, CENP-E, MCAK or HSET together with Hec1 after cold treatment. Mitotic HeLa cells treated with the indicated siRNAs were incubated on ice for 0 or 5 min before fixation and staining with anti-α-tubulin. Scale bar, 5 μm. ( d ) Quantification of microtubule signals in the middle of the spindle. The α-tubulin signal intensities in the middle region of a three-way split spindle as schematized were measured and the relative values at 5 min on ice are indicated in a bar graph. ( e ) Distribution of EB1 in cells depleted of MCAK or HSET together with Hec1. Mitotic HeLa cells were stained with anti-EB1 (green) and anti-α-tubulin (magenta). DNA was stained with DAPI (blue). All panels represent a single Z-section. Scale bar, 5 μm. ( f ) Number of EB1 dots per cell. The graph shows average number of EB1 dots in each cell. ( g ) Quantification of the microtubule signal per cell. The graph shows relative intensity of α-tubulin signal in each cell. ( h , i ) The number of EB1 dots ( h ) and the intensity of EB1 signals ( i ) were compared after adjustment by relative microtubule signal intensity in g . For the graphs in d and f – i , error bars represent the s.d. of three independent experiments measuring 10 cells each. P values were obtained by Student’s t -test. NS, not statistically significant. Full size image The contribution of Kid to chromosome congression in mammalian cells has been unclear [8] , [9] , [11] , [12] . We show that Kid is involved in chromosome motion towards the spindle equator in Hec1-depleted cells. We confirmed the depletion of Hec1 to the level where cells cannot maintain the spindle assembly checkpoint, which is only achieved after extensive depletion of Hec1 (ref. 18 ). In this condition, most of the kinetochores showed lateral attachment, and end-on attachment was rarely seen. It is probable that Hec1 is dispensable for lateral attachment, although we cannot rule out the possibility that residual Hec1 is involved in lateral attachment, as shown in budding yeast [29] . Our data suggest that Kid is involved in congression of chromosomes forming lateral attachments ( Fig. 6 ). However, does Kid play a role in chromosome congression in physiological conditions, and if so, why are congression defects not evident in Kid-depleted cells? In Kid-depleted cells, chromosome congression is probably achieved through end-on attachment by establishing bi-orientation, as previously postulated [30] . It was proposed that a NuMA-dependent traction fiber-based mechanism that pulls end-on-attached chromosomes to the spindle equator works in parallel with Kid-mediated PEFs [12] . Although such an alternative mechanism seems to compensate for the absence of Kid, it takes more time to align chromosomes, suggesting that congression through lateral attachment is more efficient than end-on attachment. It is intuitive that chromosomes close to one spindle pole are difficult to form end-on attachment with microtubules from another distant spindle pole. 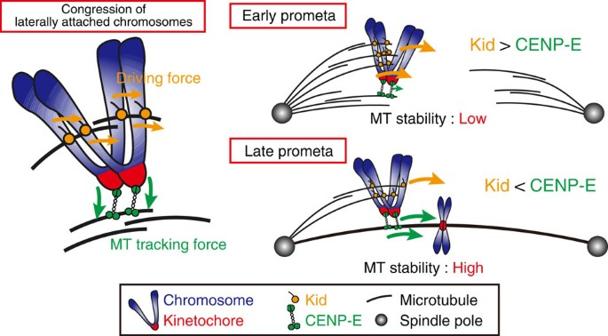Figure 6: A model for congression of laterally attached chromosomes. Left: when end-on attachment formation is perturbed by Hec1 depletion, Kid-mediated PEFs (orange arrows) drives laterally attached chromosomes towards the spindle equator, whereas CENP-E suppresses chromosome congression by causing kinetochores to track short, unstable microtubules (green arrows). Upper right: in early prometaphase, when the proportion of stabilized microtubule is small, CENP-E cannot effectively work as a motor, and Kid preferentially contributes to chromosome congression. Lower right: in late prometaphase, when the stabilized microtubules are increased, CENP-E shows high processivity and plays a predominant role in the congression of laterally attached chromosomes. See the text for more details. Figure 6: A model for congression of laterally attached chromosomes. Left: when end-on attachment formation is perturbed by Hec1 depletion, Kid-mediated PEFs (orange arrows) drives laterally attached chromosomes towards the spindle equator, whereas CENP-E suppresses chromosome congression by causing kinetochores to track short, unstable microtubules (green arrows). Upper right: in early prometaphase, when the proportion of stabilized microtubule is small, CENP-E cannot effectively work as a motor, and Kid preferentially contributes to chromosome congression. Lower right: in late prometaphase, when the stabilized microtubules are increased, CENP-E shows high processivity and plays a predominant role in the congression of laterally attached chromosomes. See the text for more details. Full size image We evaluated the distribution of kinetochores around the spindle equator in fixed cells as an index for the efficiency of chromosome congression. It is not a direct measurement of chromosome motion, but the results correlated well with that of chromosome motion. As we can measure the distance to the spindle equator for all the kinetochores in a cell, we consider this is a reliable method, although it may underestimate the efficiency of chromosome congression because the timing of cell fixation is not necessarily when the average kinetochore to spindle equator distance is minimal. Our data show that CENP-E plays an inhibitory role in chromosome congression in Hec1-depleted cells ( Fig. 6 ). This is a surprising result considering its role in the congression of chromosomes remaining around spindle poles in late prometaphase [9] . We reasoned that CENP-E cannot efficiently walk along unstable, less-bundled microtubules in the absence of stabilized kinetochore fibres, rather it works as a microtubule tip-tracker on short or depolymerizing microtubules. Depletion of MCAK or HSET facilitates the role of CENP-E on chromosome congression, probably by increasing microtubule density around the spindle equator through different mechanisms. It is unknown whether such an inhibitory function of CENP-E works in physiological conditions, but the formation of kinetochore fibres supposedly masks the effect. Our data propose the differential contribution of Kid and CENP-E to congression of laterally attached chromosomes, depending on the stability of microtubules, which may reflect the physiological situation during prometaphase. There are two microtubule populations in the spindle, discriminated by their half-lives [31] . The microtubules with longer half-lives are assumed to correspond to kinetochore microtubules, which are forming end-on attachments. It is plausible that the ratio of end-on to lateral attachment increases during prometaphase due to conversion from lateral to end-on attachment. Kinetochore microtubules themselves become further stabilized during prometaphase to metaphase [32] . Although it is currently unknown whether microtubules forming lateral attachment are somehow stabilized, we can envisage that the population of stabilized microtubules increases during prometaphase. Therefore, in early prometaphase when the proportion of stabilized microtubules is small, Kid drives chromosomes to the spindle equator while CENP-E enables kinetochores to track spindle microtubules ( Fig. 6 ). In late prometaphase, when stabilized microtubules are increased, CENP-E determines the kinetochore motion to the spindle equator ( Fig. 6 ). The contribution of Kid may also be affected by the reduction in microtubules radiating outside of the spindle during prometaphase. Chromosome congression is achieved by a cooperation of multiple mechanisms. Dynein is a minus-end-directed motor localizing to kinetochores, which is involved in rapid poleward motion of laterally attached chromosomes [33] , [34] , [35] , [36] , and implicated in chromosome congression [37] . It is not clear how CENP-E and dynein, kinetochore motors that move in opposite directions, coordinately work in chromosome congression. Kif4A is another chromokinesin belonging to the kinesin-4 family, and is suggested to play a role in chromosome congression by suppressing microtubule dynamics [8] , [9] . On meiotic chromosomes in Drosophila melanogaster , NOD, a non-motile kinesin-10, is suggested to push the chromosome arms towards the spindle equator by binding to polymerizing microtubule plus-ends [38] , [39] , [40] . End-on attachment contributes not only to chromosome motion towards the spindle equator, but also to maintaining chromosome oscillation around the spindle equator, which is dependent on Kif18A [8] . Alignment of chromosomes to the spindle equator is a prerequisite for faithful chromosome segregation, and even a subtle defect can cause chromosomal instability, which is commonly seen in cancer cells [41] . Further studies are needed for a comprehensive understanding of how chromosome alignment is achieved through differential mechanisms working on laterally and end-on-attached chromsosomes [42] . Plasmids and antibodies Monoclonal mouse antibodies against the following proteins were used: anti-Hec1 9G3 (Abcam, ab3613) for WB 1:2,000, for IF 1:1,000; anti-α-tubulin B-5-1-2 (Sigma, T5168) IF 1:3,000; anti-EB1 clone 5/EB1 (BD Bioscience, 610534) IF 1:1,000; anti-myc 9E10, WB 1:2,000, IF 1:1,000; and anti-CENP-E 1H12 (Abcam, ab5093) IF 1:1,000. Anti-Kid (Cytoskeleton Inc., AKIN12) WB 1:1,000, IF 1:500; anti-CENP-E (Sigma, C7488) WB 1:2,000, IF 1:1,000; anti-KIF2C (anti-MCAK, Abnova, H00011004-D01P) WB 1:2,000; anti-KIFC1 (anti-HSET, Sigma, HPA055997) WB 1:2,000; anti-α-tubulin (Abcam, ab18251) IF 1:3,000; and anti-GFP (Life Technologies, A11122) WB 1:3,000, IF 1:2,000 polyclonal rabbit antibodies were also used. Anti-actin I-19 (Santa Cruz, sc-1616) WB 1:5,000 polyclonal goat antibody was also used. We also used a human auto-antiserum against centromeric antigen (a gift from T. Hirota, IF 1:3,000). The pME-myc–Kid wild-type and rigor mutant (threonine134 to asparagine mutant) were gifts from M. Ohsugi [43] , [44] . The pcDNA5/FRT/TO-mycGFP–CENP-E wild-type and rigor mutant (threonine93 to asparagine mutant) were gifts from D.W. Cleveland [24] . RNA interference RNA oligonucleotides targeting complementary DNAs for Kid and HSET, and 3′ UTR for CENP-E were 5′-AAGATTGGAGCTACTCGTCGTTT-3′ (ref. 43 ), 5′-TCAGAAGCAGCCCTGTCAATT-3′ (ref. 2 ) and 5′-CCACTAGAGTTGAAAGATATT-3′ (ref. 24 ), respectively (J-Bios). A RNA oligonucleotide targeting 3′ UTR for HSET was 5′-CATGTCCCAGGGCTATCAAATTT-3′ (ref. 2 ) (J-Bios). The targeted sequences for Hec1 and MCAK were 5′-TTAATTTCTGGTCAAGAATGGCTGA-3′ and 5′-AATTGGAGTTGGCAAATGTCTGCCC-3′, respectively (Stealth, Invitrogen). For control siRNA, Stealth RNAi siRNA negative control med GC duplex #2 was used (Invitrogen). RNA duplexes (50 nM) were transfected into cells using Lipofectamine RNAiMAX reagent (Invitrogen). Cell culture and synchronization HeLa Kyoto (HeLa), HCT116 and RPE-1 cells were grown at 37 °C in a 5% CO 2 atmosphere in Dulbecco’s modified Eagle’s medium (Life Technologies), supplemented with 10% fetal bovine serum. For RNAi experiments, cells were transfected with siRNAs for 12 h and then synchronized by thymidine treatment (2 mM) for 24 h. In rescue experiments, RNAi-refractory constructs were transfected into cells with FuGENE HD (Promega) for 24 h before addition of thymidine, and cells were treated with thymidine for 24 h. In the rescue experiment for depletion of CENP-E, tetracycline (1 μg ml −1 ) was added together with thymidine. At 10 h after release from the thymidine block, synchronized mitotic cells were harvested for further analysis. Immunofluorescence analysis Cells were grown on a glass coverslip and fixed with methanol at −20 °C for 5 min. In Supplementary Figs 1 and 2b,c , cells were fixed with 1% glutaraldehyde in PHEM buffer (60 mM PIPES, 25 mM HEPES, 10 mM EGTA and 2 mM MgCl 2 ) for 10 min, and quenched with 0.1 g ml −1 NaBH 4 in PHEM for 10 min. Fixed cells were incubated with primary antibodies for 1 h, washed with PBS (137 mM NaCl, 2.7 mM KCl, 10 mM Na 2 HPO 4 and 1.8 mM KH 2 PO 4 , pH 7.4) supplemented with 0.02% Triton X-100 and incubated with secondary antibodies coupled with Alexa-Fluor-488/568 (Invitrogen, 1:2,000) for 1 h. Antibody incubations were performed in PBS supplemented with 0.02% Triton X-100. After final washes, cells were mounted with ProLong Gold (Life Technologies). Z-image stacks were captured in 0.2-μm increments on an Olympus IX-71 inverted microscope (Olympus) controlled by DeltaVision softWoRx (Applied Precision) using × 100 1.40 numerical aperture (NA) Plan Apochromat oil objective lens (Olympus). Deconvolution was performed when necessary. Image stacks were projected and saved as Photoshop files. In Supplementary Fig. 2b,c , magnified image stacks were projected with 5–7 Z-sections. In Fig. 5f–i , image stacks were projected per five Z-sections and used for quantification. All cells analysed were selected from non-overlapping fields. Each experiment was successfully repeated at least three times. Western blotting Cells were lysed in TNE-N (1% NP-40, 100 mM NaCl, 10 mM Tris-HCl, pH 7.5 and 1 mM EDTA) buffer. Protein concentration of cell lysate was measured using the Bio-Lad Protein assay kit (Bio-Rad). Cell lysates were boiled for 10 min with 4 × NuPAGE LDS sample buffer (Life Technologies). Proteins were separated by NuPAGE SDS-gel system (Life Technologies), electroblotted onto a polyvinylidene difluoride membrane (Amersham Hybond-P, GE Healthcare) and subjected to immunodetection using appropriate primary antibodies. Blocking and antibody incubations were performed in 3% non-fat dry milk. Proteins were visualized using horseradish peroxidase-labelled secondary antibodies (Santa Cruz Biotechnology, 1:3,000) and enhanced chemiluminescence, according to the manufacturer’s instructions (GE Healthcare). Uncropped versions of western blots are presented as Supplementary Fig. 8 . Live cell imaging HeLa cells expressing EGFP–α-tubulin, EGFP–CENP-A and H2B–mCherry were grown in glass chambers (Thermo). One hour before imaging, the medium was changed to pre-warmed Leibovitz’s L-15 medium (Life Technologies) supplemented with 20% fetal bovine serum and 20 mM HEPES, pH 7.0. Recordings were made in a temperature-controlled incubator at 37 °C. In Fig. 1d,e , Z-series of five sections in 3-μm increments were captured every 2 min. Image stacks were projected. In Fig. 2b,c , and Supplementary Fig. 3 , an off-axis illumination mode was used, and sections of 15 μm thickness were captured every 5 s. In Supplementary Fig. 2a , Z-series of five sections in 3-μm increments were captured every 10 min. Kinetochore motions were tracked in deconvolved movies using the StackReg [45] and Manual Tracking ( http://rsb.info.nih.gov/ij/plugins/track/track.html , F.P. Cordeliéres) plug-ins for ImageJ (NIH). All time-lapse images were collected with an Olympus IX-71 inverted microscope (Olympus) controlled by DeltaVision softWoRx (Applied Precision) using a × 20 0.75 NA UPlan SApochromat objective lens (Olympus) ( Fig. 1d,e ; Supplementary Fig. 2a ) or a × 100 1.40 NA Plan Apochromat oil objective lens (Olympus) ( Fig. 2b,c ; Supplementary Fig. 3 ). Statistical analysis Mann–Whiteney U -test was used for comparison of dispersion, and a two-sided t -test was used for comparison of average. Dispersibility of each category was validated by a two-sided F-test before the Student’s t -test. If the result of the F-test was an unequal variance, significant difference between samples was validated by a two-sided Welch’s t -test. Samples for analysis in each data set were acquired in the same experiment, and all samples were calculated at the same time for each data set. How to cite this article: Iemura, K. and Tanaka, K. Chromokinesin Kid and kinetochore kinesin CENP-E differentially support chromosome congression without end-on attachment to microtubules. Nat. Commun , 6:6447 doi: 10.1038/ncomms7447 (2015).